Observation of the nonlocal spin-orbital effective field The spin-orbital interaction in heavy nonmagnetic metal/ferromagnetic metal bilayer systems has attracted great attention and exhibited promising potentials in magnetic logic devices, where the magnetization direction is controlled by passing an electric current. It is found that the spin-orbital interaction induces both an effective field and torque on the magnetization, which have been attributed to two different origins: the Rashba effect and the spin Hall effect. It requires quantitative analysis to distinguish the two mechanisms. Here we show sensitive spin-orbital effective field measurements up to 10 nm thick ferromagnetic layer and find the effective field rapidly diminishes with the increase of the ferromagnetic layer thickness. We further show that this effective field persists even with the insertion of a copper spacer. The nonlocal measurement suggests that the spin-orbital effective field does not rely on the heavy normal metal/ferromagnetic metal interface. Spin transfer torque, which was conventionally generated by a spin-polarized current, has become a useful tool to manipulate magnetizations [1] , [2] , [3] , [4] . A more effective and robust spin transfer torque can be realized through the diffusion of a pure spin current, where charge transfer is eliminated [5] , [6] , [7] . The spin Hall effect (SHE) has been proposed as a convenient source to generate a pure spin current in order to manipulate magnetization for information recording and data processing [8] , [9] , [10] , [11] , [12] . It has been experimentally demonstrated that the pure spin current generated from the SHE can affect magnetic fluctuation [13] , relaxation time of magnetization dynamics [14] , [15] , [16] and magnetization switching [17] . In these experiments, the sample under test is usually a double-layered thin film composed of a heavy nonmagnetic metal layer (HM) to generate spin current via the SHE and a ferromagnetic layer (FM) to manifest the effect of the spin current. The response of the ferromagnetic layer is assumed to follow Slonczewski’s model [18] , [19] , in which the magnetization dynamics is described by a modified Landau–Lifshitz–Gilbert equation with an additional torque term, that is, Slonczewski torque, due to the spin current generated from the SHE. Though often considered negligible in the spin transfer torque effect, it is theoretically predicted that the spin current can also generate an effective field when the FM layer is very thin [20] , [21] . The simple picture of the spin Hall process is illustrated in Fig. 1a . Under an electric bias, electrons with different spins separate in the HM and diffuse into the adjacent FM due to the SHE. The spins dephase due to the exchange interaction with the FM with respect to its own momentum and the transverse magnetic moment averages out to be zero if the FM is thicker than a characteristic spin dephasing length. However, if the FM is thin enough that the transverse moment is not fully randomized, the spins will also generate an out-of-plane torque or an in-plane effective field onto the FM layer. This field-like term was reported in spin transfer torque in magnetic tunnel junctions, but was rarely observed in metallic spin valves [22] , [23] . 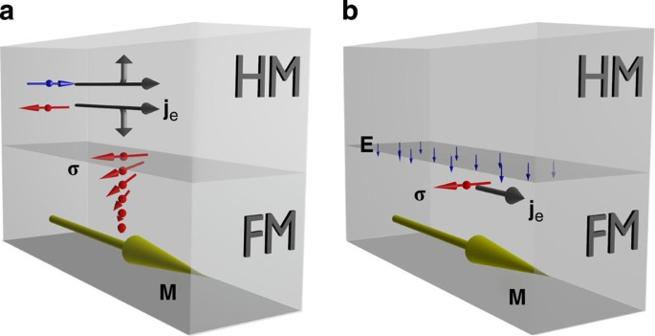Figure 1: Sketches of two mechanisms for spin orbital torque and field. (a) SHE: electric current through the HM layer generates a spin current via SHE. The spin current exerts an effective torque and field on the adjacent FM layer via the spin transfer effect. (b) Rashba effect: an electric current through the interface between HM and FM layer experience a Rashba field via the spin-orbital interaction under the structural inversion asymmetry. Through the exchange coupling and spin relaxation, the Rashba effect exerts an effective field as well as a torque on the FM. Figure 1: Sketches of two mechanisms for spin orbital torque and field. ( a ) SHE: electric current through the HM layer generates a spin current via SHE. The spin current exerts an effective torque and field on the adjacent FM layer via the spin transfer effect. ( b ) Rashba effect: an electric current through the interface between HM and FM layer experience a Rashba field via the spin-orbital interaction under the structural inversion asymmetry. Through the exchange coupling and spin relaxation, the Rashba effect exerts an effective field as well as a torque on the FM. Full size image On the other hand, it is proposed lately that the Rashba effect can also generate a Slonczewski-like torque [24] , [25] as well as an effective field [26] , [27] , [28] . The Rashba effective field was first reported in 2D electron gas in semiconductors [29] and later in metallic systems [30] . The effective torque and field arise from the spin-orbital interaction at the HM/FM interface under structural inversion asymmetry as illustrated in Fig. 1b , while the SHE takes place inside the HM layer. However, the effects on magnetization dynamics from the Rashba effect and the SHE are very similar. In this manuscript, we report the observation of an effective field generated by the spin-orbital interaction in a HM/FM bilayer film, and show that this effective field can be generated nonlocally even with a Cu layer inserted in between, which suggests the HM/FM interface is not necessary for the spin-orbital effective field (SOF). We also show that this effective field has unique thickness dependences, and has an important role in the current induced magnetization switching [31] . Detection of the SOF Despite the different possible physical origins, an electric current through a HM/FM bilayer produces two types of torques on the magnetization of FM: a field-like term and a torque-like term , where is the magnetization, is a unit vector in the film plane and perpendicular to the d.c. current, and a , b are parameters related to the excitations [32] . We used a d.c. planar Hall measurement geometry to investigate the magnitude of the SOF in HM/FM bilayers. We prepared samples of Ni 80 Fe 20 /Cu, Ni 80 Fe 20 /Pt and Ni 80 Fe 20 /Ta with various thicknesses and spacer layers. The samples were patterned as a Hall bar as shown in Fig. 2a . 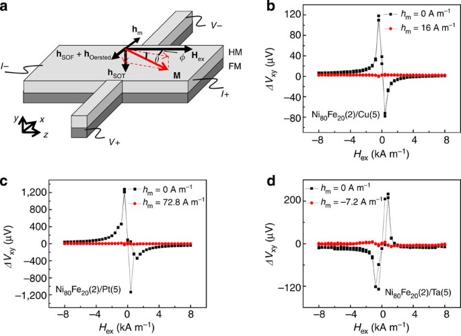Figure 2: Observation of the SOF. (a) Planar Hall structure to detect the magnetization reorientation. The Hall bar is 1 mm wide and 1 cm long. (b–d) In these graphs, the second order PHE voltage are measured at 50 mA bias for Ni80Fe20(2)/Cu(5) and Ni80Fe20(2)/Pt(5) and at 10 mA bias for Ni80Fe20(2)/Ta(5) due to its high resistivity, respectively. The voltage signals without cancellation field are shown in black curves and those after cancellation field are shown in red curves. Transverse voltage V xy was detected, which consists of both the planar Hall effect (PHE) signal and the anomalous Hall effect (AHE) signal, Figure 2: Observation of the SOF. ( a ) Planar Hall structure to detect the magnetization reorientation. The Hall bar is 1 mm wide and 1 cm long. ( b – d ) In these graphs, the second order PHE voltage are measured at 50 mA bias for Ni 80 Fe 20 (2)/Cu(5) and Ni 80 Fe 20 (2)/Pt(5) and at 10 mA bias for Ni 80 Fe 20 (2)/Ta(5) due to its high resistivity, respectively. The voltage signals without cancellation field are shown in black curves and those after cancellation field are shown in red curves. Full size image where w is the width of the Hall bar strip, j is the d.c. current density, Δ ρ is the anisotropic resistivity defined as the resistivity difference between the longitudinal and transverse magnetization configurations, ρ AHE is the anomalous Hall resistivity, M x , M y , M z are the magnetizations in the x , y , z direction, respectively, and M s is the saturation magnetization. In a stationary state with saturated magnetization, the PHE arises from the in-plane magnetization component, which is primarily due to the competition among the external field, magnetic anisotropy and the effective field generated by the current. The AHE is due to the out-of-plane magnetization component, which is driven by the spin-orbital effective torque (SOT) generated by the current. Here we note that, in the first order approximation, the SOT can be viewed as an out-of-plane effective field , where γ is the gyromagnetic ratio. Therefore, the contribution of the SOT to the in-plane magnetization rotation is neglected (see Supplementary Note 1 ). For a 10 10 A m −2 current density through a 5-nm Pt in a Ni 80 Fe 20 (2)/Pt(5) bilayer (the numbers in parentheses are thicknesses in nanometres), we estimate that the magnetization only tilts 0.015° out of plane due to the SOT. On the other hand, this amount of current can generate a 25-A m −1 magnetic field in the x direction due to Ampere’s Law, which results in a 0.6° magnetization reorientation in the film plane under a 2.4-kA m −1 d.c. saturation field in the z direction. Owing to the similar order of magnitude of ρ AHE (0.9 Ω nm −1 ) with Δρ (0.4 Ω nm −1 ), the AHE voltage is much smaller compared with the PHE voltage according to Equation (1) (see Supplementary Notes 1–3 ). Therefore, by neglecting the AHE voltage contribution, the detected transverse voltage signal is , where the in-plane magnetization direction is a function of external magnetic field H ex and further changes with the current induced in-plane effective field h I , . The h I may include both an Oersted field and a spin orbital effective field . It is convenient to use the second order term, by adding V xy at both positive and negative current bias to highlight the contribution of the current induced magnetization reorientation [33] . Here, we expect the current induced effective field to be linearly proportional to the current density that is a constant. In a simplified scenario, when the easy axis of magnetic anisotropy is along the z direction and the magnetization is saturated by H ex , the current induced effective field h I in the x direction causes the magnetization to rotate from to , where H eff includes H ex and anisotropy fields. As a result, the second order transverse voltage ΔV xy is inversely proportional to H eff under a reasonable assumption that h I is much smaller than H eff . In order to show the current induced effective field includes both an Oersted field and an effective field due to the spin-orbital interaction, three samples of Ni 80 Fe 20 (2)/Cu(5), Ni 80 Fe 20 (2)/Pt(5) and Ni 80 Fe 20 (2)/Ta(5) are measured. Copper is one of the most popular materials that has been used as a reference with weak spin-orbital interaction and a long spin diffusion length [34] . Therefore, in the first sample, as shown in Fig. 2b , the measured Δ V xy is solely due to the Oersted field generated by the applied d.c. current. In Fig. 2c , the Δ V xy for Ni 80 Fe 20 /Pt sample shows a much enhanced signal even though the sheet resistance and anisotropic magneto resistance are similar to those of the Ni 80 Fe 20 /Cu sample. The SOF in the Ni 80 Fe 20 /Pt sample is in the same direction as the current induced Oersted field. Furthermore, shown in Fig. 2d , the Δ V xy for Ni 80 Fe 20 /Ta sample shows a reversed profile indicating the d.c. current generates an SOF in the opposite direction of the Oersted field, which is consistent with the opposite spin Hall angles in Ta and Pt layers [17] , [35] , [36] . Directly extracting the magnitude of the effective field h I from Δ V xy requires a calibration of resistivity, anisotropy profile and anisotropic magneto resistance. Instead we use a secondary Helmholtz coil, which applies a cancellation magnetic field h m parallel to the effective field generated by the current. The second order PHE voltage ΔV xy is obtained by adding the PHE voltage at positive and negative bias currents along with simultaneously reversed h m . Therefore, if the cancellation magnetic field h m matches the current induced effective magnetic field h I , the measured shall vanish. Indeed, such cancellation can be achieved as shown in Fig. 2b–d . The fact that the transverse voltage can be almost completely cancelled out by the applied d.c. magnetic field further confirms that the measured voltage signal is due to the field-like term. Other potential artifacts regarding misalignment of the external magnetic field, proximity effect in Pt, thermal effect and so on are ruled out as detailed in Supplementary Note 2 . The cancellation magnetic field is equal to the superposition of the Oersted field and the SOF. As Cu has a negligible spin-orbital interaction, the 16.0 A m −1 cancellation field in Ni 80 Fe 20 (2)/Cu(5) only corresponds to the Oersted field. The cancellation field of Ni 80 Fe 20 (2)/Pt(5) is 72.8 A m −1 , which is much greater than the 25.0 A m −1 Oersted field due to Ampere’s Law even if we assume all the current flows through Pt. The SOF has opposite direction for the Ni 80 Fe 20 /Ta sample. Characterization of the SOF In most of the previous experiments, the HM is in direct contact with the FM, leading to the ambiguity of bulk effect in the HM due to the SHE and interface effect at the HM/FM interface due to the Rashba effect. In order to study the importance of the HM/FM interface for the SOF, we further measured the SOF for Ni 80 Fe 20 (2)/Pt(5) with a copper spacer layer. As shown in Fig. 3a , the magnitude of the SOF in the samples with up to 4 nm Cu spacer layer is still higher than 25.0 A m −1 , which is the maximum possible Oersted field estimated by assuming all current flows through Pt. However, as the current is partially shorted by Ni 80 Fe 20 , a more plausible comparison is with the Oersted fields generated in control samples Ni 80 Fe 20 (2)/Cu( x ) with similar sheet resistance. It is observed that the SOF does not vanish even with the insertion of 8 nm Cu. Spin current is generally considered to be dissipationless in Cu. One apparent cause for the reduction of the SOF is that the current is shorted by the Cu spacer layer, which has a higher conductivity than that of Pt. The total current induced field is , where j Pt is the current density through Pt, and β is the coefficient that describes the strength of the SOF. Although the current density j Pt cannot be accurately determined as the resistivity of Cu, Ni 80 Fe 20 and Pt may vary with the thickness of Cu due to morphology change and interface scattering [37] , [38] , it is reasonable to argue that the reduction of the SOF is because j Pt decreases with the insertion of Cu. The nonlocal measurement indicates that the HM/FM interface is not necessary for the SOF, which can be qualitatively explained with the spin current transfer torque generated from the SHE. However, this suggests a longer spin dephasing length than theoretical predictions where the spin dephasing length is expected to be only several atomic layer thick [3] . One may also argue that a nonlocal spin current can be generated at the Pt/Cu interface via Rashba effect. However, regardless of the origin of the spin current, our result suggests that the spin transfer torque generated by the nonlocal spin current is one important mechanism in the SOF. Here, we would like to point out that our experiment does not exclude the possible existence of the Rashba effective field when Ni 80 Fe 20 is in direct contact with Pt. 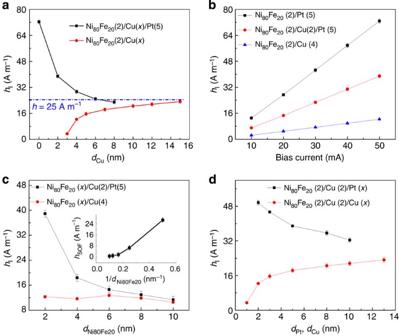Figure 3: Quantitative determination and characterization of the SOF. (a) Under a 50-mA bias, the current induced effective field in Ni80Fe20(2)/Cu(x)/Pt(5) (black dots, the line is for guide of eyes) decays with the increase of the Cu spacer layer thickness. The maximum possible Oersted field is 25 A m−1(blue dashed line). The red curve shows the Oersted field in control samples of Ni80Fe20(2)/Cu(x). An exemplary extraction of thehIand the error is shown inSupplementary Fig. S1. (b) The current induced effective field has a linear dependence with the bias current. (c) When the Ni80Fe20thickness increases, the current induced effective field in Ni80Fe20(x)/Cu(2)/Pt(5) (black) quickly reaches the Oersted field generated in reference samples of Ni80Fe20(x)/Cu(4) with similar sheet resistances (red). The inset shows the thickness dependence of the SOF that deviates from 1/dNi80Fe20. The bias current is 50 mA. (d) The Oersted field increases with increasing normal metal layer thickness in the control sample of Ni80Fe20(2)/Cu(2)/Cu(x) (red). However, the total current induced effective field in Ni80Fe20(2)/Cu(2)/Pt(x) decreases with increasing Pt thickness (black). The bias current is 50 mA. Figure 3: Quantitative determination and characterization of the SOF. ( a ) Under a 50-mA bias, the current induced effective field in Ni 80 Fe 20 (2)/Cu( x )/Pt(5) (black dots, the line is for guide of eyes) decays with the increase of the Cu spacer layer thickness. The maximum possible Oersted field is 25 A m −1 (blue dashed line). The red curve shows the Oersted field in control samples of Ni 80 Fe 20 (2)/Cu( x ). An exemplary extraction of the h I and the error is shown in Supplementary Fig. S1 . ( b ) The current induced effective field has a linear dependence with the bias current. ( c ) When the Ni 80 Fe 20 thickness increases, the current induced effective field in Ni 80 Fe 20 ( x )/Cu(2)/Pt(5) (black) quickly reaches the Oersted field generated in reference samples of Ni 80 Fe 20 ( x )/Cu(4) with similar sheet resistances (red). The inset shows the thickness dependence of the SOF that deviates from 1/ d Ni80Fe20 . The bias current is 50 mA. ( d ) The Oersted field increases with increasing normal metal layer thickness in the control sample of Ni 80 Fe 20 (2)/Cu(2)/Cu( x ) (red). However, the total current induced effective field in Ni 80 Fe 20 (2)/Cu(2)/Pt( x ) decreases with increasing Pt thickness (black). The bias current is 50 mA. Full size image Both the Oersted field and the SOF are proportional to the bias current. The linear dependence of the total current induced effective fields with the bias current is confirmed in Fig. 3b . Here, the maximum current density through the bilayer is <10 10 A m −2 . No significant thermal effect is observed. This also indicates that the operation condition is in the linear response regime, where complication due to nonlinear SOT effect does not occur. The current induced field in a Ni 80 Fe 20 (2)/Cu(4) is only due to Ampere’s Law, and therefore, the ratio between the current and its generated field is calculated as . We make a rough assumption that the current through Cu in the Ni 80 Fe 20 (2)/Cu(4) bilayer is the same as that through Pt in the Ni 80 Fe 20 (2)/Pt(5) bilayer because the sheet resistance of the two bilayers are similar, . Therefore, the SOF coefficient can be extracted to be . The value of the SOF coefficient may contain error due to the estimation on j Pt . A more accurate determination of current distribution for this thin bilayer system should be using Fuchs–Sondheimer model with knowledge of spin-dependent conductivity in Ni 80 Fe 20 as well as the interface scattering coefficient [39] , which is difficult to carry out. However, we can set a lower bound of the SOF coefficient by assuming that all current flows through Pt, leading to a 10 10 A m −2 current density in Pt. The lower bound of the SOF coefficient for Ni 80 Fe 20 (2)/Pt(5) is calculated as 4.8 nm. Similarly, by assuming the −7.2 A m −1 total effective field is due to all the 10 mA current through Ta in the Ni 80 Fe 20 (2)/Ta(5), we can also set the lower bound of the SOF coefficient of Ni 80 Fe 20 (2)/Ta(5) to be – 6.1nm. As a comparison, the coefficient of the Slonczewski torque-like term is calculated to be 11.5 nm for Pt and −16.0 nm for Ta by using following Liu’s argument, where σ SH is the spin Hall angle of the HM (0.07 for Pt and −0.1 for Ta), μ 0 M s =1 T, and d FM is the thickness of the FM [17] , [19] . It is theoretically predicted that the SOF is sensitive to the magnetic layer thickness [32] . The magnetic layer thickness dependence shown in Fig. 3c indicates that the SOF decays quickly as the magnetic layer thickness increases. We estimate the SOF by subtracting the Oersted field of control samples with similar sheet resistance h SOF ( x ) = h I [Ni 80 Fe 20 ( x )/ Cu (2)/ Pt (5)] – h I [Ni 80 Fe 20 ( x )/ Cu (4)]. As indicated in the inset of Fig. 3c , the decaying rate is faster than 1/ d Ni80Fe20 dependence, which is qualitatively consistent with theoretical predictions with SHE [32] . The magnitude of the SOF decays with the Pt thickness when the same amount of current passes through it due to the reduction of current density in Pt and/or at the Pt/Cu interface. On the other hand, the total current through the normal metal reduces with the reduction of normal metal thickness, which results in a lower Oersted field. This is confirmed in Fig. 3d , where opposite trends of current induced effective field are observed between Ni 80 Fe 20 (2)/Cu(2)/Pt( x ) and the control sample Ni 80 Fe 20 (2)/Cu(2)/Cu( x ). SOF induced magnetization switching It has been demonstrated that the SOT can switch magnetization efficiently, which may benefit the potential application in magnetic random access memory [17] , [31] . Also inherited from the spin-orbital interaction, the SOF is an in-plane effective field that also facilitates magnetization switching. Here, we show that the SOF can indeed switch magnetization by performing a similar planar Hall measurement. The detection structure is shown in Fig. 4a , with an elliptical dot of Ni 80 Fe 20 (2)/Ta(1) lithographically patterned on a 5-nm thick Pt strip. The easy axis of the sample is purposely set about 10° off the external magnetic field and the transverse resistance R xy = V xy / I is measured in order to indicate magnetization reorientation as well as magnetization reversal. As shown in Fig. 4b , the sharp transition in the transverse resistance curve is associated with magnetization reversal due to the change of the field from H ex + H an to H ex − H an ( [40] ). The SOT-induced magnetization reversal is suppressed here as the damping of Ni 80 Fe 20 is >0.05 due to the spin-pumping effect [41] . As revealed in Fig. 4b , not only the reversal field is shifted when current is applied, but also the magnetization reorientation at saturated field is shifted the same amount. This can only be explained with an effective field rather than the SOT. 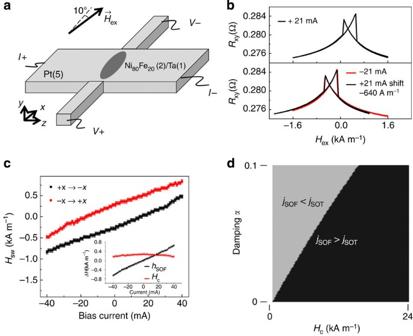Figure 4: The SOF induced in-plane magnetization switching. (a) Experimental setup for the SOF-induced magnetization reversal. The width of the Hall bar is 50 μm. The magnetic film is patterned into a 40 × 20 μm2elliptical dot. (b) Magnetization reversal can be revealed from the sharp transition in the transverse resistance. The switching fields shift toward two opposite directions when applied+21 mA and −21 mA bias current. When the curve corresponding to +21 mA is shifted −640 A m−1along thexaxis, the two curves overlap, indicating that the shift of magnetization reversal and reorientation have the same origin from the SOF. The magnitude of current induced effective field is consistent with the same sample measured using the Hall bar as shown in Fig. 2a, but is smaller than that in the Ni80Fe20(2)/Pt(5) as shown in Fig. 2c. We attribute this to the film conductivity difference in different film growth sequence. The current through Pt is smaller in Pt(5)/ Ni80Fe20(2)/Ta(1) than that in Ni80Fe20(2)/Pt(5). (c) The magnitude of the switching field changes monotonically with the bias current. The two curves are subtracted to determine the coercivity field as shown in the red curve in the inset. Owing to thermal heating, the coercivity reduces at high current bias. When the two curves are averaged, the switching field due to the thermally driven coercivity change is removed. Here, the tolerances of the extracted switching fields equal to the swept field step due to the sharp magnetization switching. (d) The comparison of magnetization switching efficiency between the SOT and the SOF is plotted by comparing the critical current density with respect to different dampings and coercivities. The parameters used areμ0Ms=1 T,μ0Meff=0.55 T,σSH=0.07,dFM=2 nm,β=12.7 nm. Figure 4c shows that the switching field shifts depending on the direction of the applied current and changes monotonically with the magnitude of the bias current. The bending of the curve is due to thermal effect at high current bias. The existence of the SOF may also partially explain the slanted current induced switching phase diagram measured in CoFeB/Ta system [17] . Figure 4: The SOF induced in-plane magnetization switching. ( a ) Experimental setup for the SOF-induced magnetization reversal. The width of the Hall bar is 50 μm. The magnetic film is patterned into a 40 × 20 μm 2 elliptical dot. ( b ) Magnetization reversal can be revealed from the sharp transition in the transverse resistance. The switching fields shift toward two opposite directions when applied+21 mA and −21 mA bias current. When the curve corresponding to +21 mA is shifted −640 A m −1 along the x axis, the two curves overlap, indicating that the shift of magnetization reversal and reorientation have the same origin from the SOF. The magnitude of current induced effective field is consistent with the same sample measured using the Hall bar as shown in Fig. 2a, but is smaller than that in the Ni 80 Fe 20 (2)/Pt(5) as shown in Fig. 2c. We attribute this to the film conductivity difference in different film growth sequence. The current through Pt is smaller in Pt(5)/ Ni 80 Fe 20 (2)/Ta(1) than that in Ni 80 Fe 20 (2)/Pt(5). ( c ) The magnitude of the switching field changes monotonically with the bias current. The two curves are subtracted to determine the coercivity field as shown in the red curve in the inset . Owing to thermal heating, the coercivity reduces at high current bias. When the two curves are averaged, the switching field due to the thermally driven coercivity change is removed . Here, the tolerances of the extracted switching fields equal to the swept field step due to the sharp magnetization switching. ( d ) The comparison of magnetization switching efficiency between the SOT and the SOF is plotted by comparing the critical current density with respect to different dampings and coercivities. The parameters used are μ 0 M s =1 T, μ 0 M eff =0.55 T, σ SH =0.07, d FM =2 nm, β =12.7 nm. Full size image In a HM/FM bilayer, a magnetization reversal due to the SOT is an anti-damping process, of which the critical current strongly depends on the damping α of the FM, while having large tolerance on the coercivity H c . The critical current density to induce magnetization switching at zero temperature is given by [17] . where M eff is the effective magnetization arisen from the demagnetization and surface anisotropy. On the other hand, the SOF-induced magnetization reversal is insensitive to the damping, but strongly depends on the coercivity. The critical current density to induce magnetization switching can be calculated as Using the parameters extrapolated in our experiment and those reported in the literature, we show in Fig. 4d the difference in magnetization reversal efficiency deploying SOT and SOF with respect to different damping and coercivity. In this second order PHE voltage measurement, we purposely chose Ni 80 Fe 20 , which has a weak anomalous Hall resistance, so that the contribution of AHE is minimized. However, for other magnetic materials with a stronger AHE signal, the SOT term can be obtained by proper analysis and line-shape fitting as discussed in Supplementary Note 3 . Several groups have measured the field-like term in similar HM/FM bilayers, but with a perpendicular anisotropy. The field-like term was estimated in AlOx/Co/Pt by Liu et al . [42] to be below their experimental detection limit, which is β <10 nm . But very recently, Garello et al . [43] showed that the SOF coefficient in similar system can be as large as 23 nm< β <54 nm through controlled annealing process. On the other hand, Kim et al . [44] showed the SOF coefficient is about 10 nm< β <30 nm in the MgO/CoFeB/Ta system. The value β ~12.7 nm extracted in our Ni 80 Fe 20 (2)/Pt(5) sample is in similar range with these experimental reports. The discrepancy is because the SOF coefficient strongly depends on the ferromagnetic material and layer thickness. The SOF in HM/FM bilayer system with in-plane anisotropy is rarely studied and was neglected in the spin torque driven ferromagnetic resonance (ST-FMR) experiments [19] . As an independent check, we have also carried out the ST-FMR experiments on Co 40 Fe 40 B 20 /Ta sample. Both the SOT and the current induced field can be extracted from the symmetric and antisymmetric rectified voltage spectra, respectively. As the SOF generated by the current has opposite direction with the Oersted field due to the sign of the spin Hall angle of Ta, the antisymmetric rectified voltage spectra should have a 180° phase change when the SOF dominates the Oersted field. Indeed, we observed the reversal of the antisymmetric voltage profile in thin CoFeB and Ta layers as shown in Fig. 5 . This result further confirms that the SOF depends on the spin Hall angle of the HM. 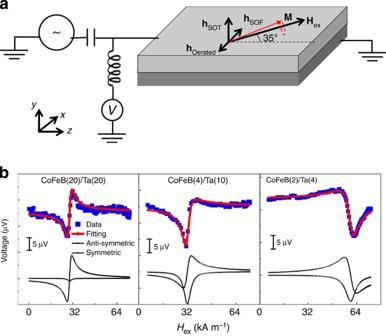Figure 5: Observation of the SOF using ST-FMR technique. (a) Experimental setup for ST-FMR measurement. (b) Measured rectified voltage (blue dot) and fitting curves (red line) for three different samples. The curves are fitted usingThe fitted anti-symmetric component and symmetric component are shown in black curves in the graph. As the films become thinner, the anti-symmetric component switches signs indicating there is an effective field that has opposite direction as the Oersted field. The microwave frequency was 7 GHz. Various microwave power from 10 to 25 dBm were used during the measurement depending on the thickness of the sample. Consistent results were observed for different microwave power and frequencies. Figure 5: Observation of the SOF using ST-FMR technique. ( a ) Experimental setup for ST-FMR measurement. ( b ) Measured rectified voltage (blue dot) and fitting curves (red line) for three different samples. The curves are fitted using The fitted anti-symmetric component and symmetric component are shown in black curves in the graph. As the films become thinner, the anti-symmetric component switches signs indicating there is an effective field that has opposite direction as the Oersted field. The microwave frequency was 7 GHz. Various microwave power from 10 to 25 dBm were used during the measurement depending on the thickness of the sample. Consistent results were observed for different microwave power and frequencies. Full size image Sample preparation The samples were deposited on silicon substrates with 1 μm thermal oxide layer via magnetron sputtering. The deposition rates were 0.27 nm s −1 (Ni 80 Fe 20 ), 0.13 nm s −1 (Cu), 0.07 nm s −1 (Pt, Ta, Co 40 Fe 40 B 20 ) in an argon pressure of 4.5 × 10 −3 Torr. After deposition, samples with Cu as the top layer were coated with 3.5 nm of SiO 2 to prevent oxidation. The growth rate of SiO 2 was 0.02 nm s −1 in an argon pressure of 2 × 10 −3 Torr with radio-frequency sputtering. Samples with Pt as the top layer were not capped with SiO 2 . The samples used for the Hall measurement were fabricated by one-step photolithography. The long axis of the Hall bar was patterned along the easy axis direction of Ni 80 Fe 20 . The samples used for the SOF-induced magnetization reversal were first patterned into a similar Hall bar, followed by a second ion beam etching to define the elliptical shaped dot. The long axis of the Hall bar was patterned along the hard axis direction of Ni 80 Fe 20. The samples used for the ST-FMR measurement were fabricated by two-step photolithography. The sample was firstly patterned into a rectangular dot with sizes ranging from 20 × 20 to 50 × 10 μm 2 to ensure the resistance is about 50 Ω for different thicknesses. A stack of conductive film Ta (10)/Cu (600)/Au (200) was then deposited to form a coplanar waveguide that guides the microwave into the sample. The coplanar waveguide has an overall length <600 μm, which is much less than the wavelength of the microwave. Measurement setup A Keithley 220 current source and a Keithley 2182A nanovolt metre were used in the Hall measurement. The external magnetic field was generated by a Helmholtz coil driven by a Kepco power supply 20–20. The cancellation magnetic field was generated by a smaller Helmholtz coil driven by a Keithley 224 current source. In the ST-FMR measurement, the microwave was generated by an Agilent E8257D signal generator and guided into the sample through a Cascade GSG-100 coplanar air probe. The d.c. rectified voltage was separated from the microwave signal using a bias Tee and measured by a Keithley 2182A nanovolt metre. The external magnetic field was generated by an electromagnet driven by a Kepco power supply 50–20. The external field was offset at an optimized angle 35° off the z axis. Extraction of the current induced in-plane effective field When the cancellation fully balances the current induced in-plane effective field h I , the second order planar Hall voltage shall vanish. The criteria of the fully balancing is determined by the s.d. of the at saturated states, , and the proper balancing state is when V sd reaches minimum. The tolerance is determined by the 3 dB points, where the V sd is twice higher than the optimized balancing. An exemplary extraction is shown in the Supplementary Fig. S1 . How to cite this article: Fan, X. et al . Observation of the nonlocal spin-orbital effective field. Nat. Commun. 4:1799 doi:10.1038/ncomms2709 (2013).